Aryl hydrocarbon receptor negatively regulates NLRP3 inflammasome activity by inhibiting NLRP3 transcription NLRP3 inflammasome is a multi-protein complex, which plays crucial roles in host defense against pathogens. The NLRP3 protein level is considered rate limiting for the activation of the inflammasome, thus its expression must be tightly controlled to maintain immune homeostasis. However, the molecular mechanisms that modulate NLRP3 expression, especially at the transcriptional level, remain largely unknown. In the present study, we show that aryl hydrocarbon receptor (AhR) activation inhibits NLRP3 expression, caspase-1 activation and subsequent IL-1β secretion in peritoneal macrophages, whereas siRNA knockdown of AhR has opposite effects. AhR could bind to the xenobiotic response element (XRE) in the NLRP3 promoter and inhibit NLRP3 transcription. Furthermore, AhR activation suppresses Alum-induced peritonitis in vivo . Therefore, we identified AhR as a negative regulator of NLRP3 inflammasome activity by inhibiting the transcription of NLRP3 and suggested AhR as a potential target for the intervention of diseases with uncontrolled inflammasome activation. NLRP3 is a crucial pattern recognition receptor and plays pivotal roles in host defense against microbial pathogens. NLRP3 assembles a multi-protein complex termed inflammasome, which comprise the following molecules-NLRP3, apoptotic speck protein containing a caspase recruitment domain (ASC) and Caspase-1 (refs 1 , 2 , 3 , 4 ). Inflammasome formation is triggered by a range of stimuli (for example, bacterial toxins including nigericin, crystals such as silica, extracellular ATP, amyloid-β and alum) that emerge during infections, tissue damage or metabolic imbalances. Once the protein complexes were formed, the inflammasomes activate of caspase-1, which then process pro-interleukin (IL)-1β and pro-IL-18 into mature IL-1β and IL-18 (refs 1 , 2 , 3 , 4 ). The NLRP3 inflammasome has been implicated in a variety of diseases, such as gout, type 2 diabetes, atherosclerosis, Alzheimer’s disease, acute graft-versus-host disease and cancers [5] , [6] , [7] . Thus, a fine balance must be maintained between the activation and inhibition of inflammasome to avoid detrimental effects. The NLRP3 protein level is critically required for inflammasome assembly and is considered as a rate-limiting element for the activation of inflammasome [8] , [9] , thus its expression must be tightly controlled to maintain immune homeostasis. In resting macrophages, the protein level of NLRP3 is relatively low, so that NLRP3 inflammasome assembly is hardly induced [9] , [10] . NLRP3 expression can be induced by exogenous and endogenous factors, including TLR agonists and proinflammatory cytokines, which further allow respective NLRP3 activators to trigger caspase-1 cleavage and subsequently IL-1β secretion. Up to now, multiple regulatory mechanisms have been identified to attenuate the NLRP3 inflammasome activation [4] , [9] , such as autophagy [11] , [12] , T cells [13] , type I interferon [14] , nitric oxide [15] , TRIM30 (ref. 16 ), LRRFIP2 (ref. 17 ) and so on. Among these regulators, several molecules are directly inhibiting NLRP3 protein expression to attenuate inflammasome activation, such as plasminogen activator inhibitor type 2 (ref. 18 ) and miR-223 (refs 19 , 20 ). Plasminogen activator inhibitor type 2 suppresses NLRP3 expression via increasing autophagy and NLRP3 degradation [18] . MiR-223 suppresses NLRP3 expression through a conserved binding site within the 3′ untranslated region of NLRP3, translating to reduced NLRP3 inflammasome activity [19] , [20] . However, all the identified regulators of NLRP3 work at the posttranscriptional level, and the transcriptional regulation of NLRP3 expression remains to be defined. To identify the potential regulator of NLRP3 at the transcription level, we analysed the murine NLRP3 promoter segment, and identified three putative aryl hydrocarbon receptor (AhR) binding sites, which indicates that AhR may play regulatory roles in the NLRP3 transcription. AhR is a ligand-dependent basic helix-loop-helix transcription factor that can be activated by a broad array of ligands, including environmental contaminants (such as dioxin and xenobiotic substances) and potential endogenous ligands (such as dietary components, hememetabolites, indigoids and tryptophan metabolites) [21] . Among these AhR ligands, 2, 3, 7, 8-tetrachlorodibenzo-p-dioxin (TCDD, a common dioxin) is recognized as one of the most potent agonist, which is widely distributed in our living environment; whereas tryptophan photoproduct 6-formylindolo-[3, 2-b]-carbazole (FICZ) is its endogenous ligand [22] , [23] . Following engagement by its cognate ligands, AhR undergoes conformation changes, translocates to the nucleus, forms a heterodimer with ARNT (AhR nuclear translocator) and binds to the xenobiotic response element (XRE) in the promoter of target genes, which causes a variety of regulatory effects [22] , [23] . Recent results highlight major roles of AhR in both adaptive and innate immune system [22] , [23] , [24] , [25] . However, the functional role of AhR in inflammasome activation has never been described. In this study, we show that AhR could bind to the XRE region located in the promoter of NLRP3, inhibit NLRP3 transcription and subsequent inflammasome activation. The identification of AhR as a physiological suppressor of NLRP3 inflammasome provides an explanation on the fine modulation of inflammasome activity under physiological conditions. AhR inhibits NLRP3 expression To investigate the possible functions of AhR on NLRP3 expression, mouse peritoneal macrophages were pretreated with TCDD, followed by stimulation with LPS (TLR4 ligand). TCDD treatment significantly attenuated LPS-induced NLRP3 expression at both protein and mRNA level ( Fig. 1a,b ). In addition, FICZ inhibited NLRP3 expression in a dose-dependent manner as well as TCDD ( Fig. 1c ). Taken together, these results indicate that AhR activation inhibits LPS-induced NLRP3 production. 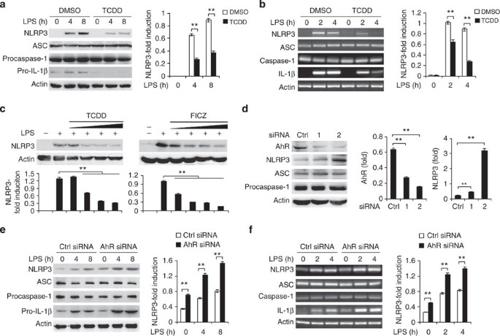Figure 1: AhR inhibits NLRP3 expression. (a,b) Mouse peritoneal macrophages were pretreated with dimethylsuphoxide (DMSO) or TCDD for 40 min and then stimulated with LPS for the indicated periods. NLRP3, ASC, caspase-1, IL1β and Actin were detected by western blot (a) and RT-PCR (b). (c) Mouse peritoneal macrophages were pretreated with increasing concentration of TCDD (2, 10, 20, 50 nM) or FICZ (20, 100, 200, 500 nM) for 40 min and then stimulated with LPS for 8 h. NLRP3 and Actin were detected by western blot. (d) Western blot analysis of NLRP3, ASC, Procaspase-1, AhR and Actin expression in mouse peritoneal macrophages transfected with scrambled control siRNA or AhR siRNA for 48 h. (e,f) Mouse peritoneal macrophages transfected with control siRNA or AhR siRNA were stimulated with LPS for the indicated periods. NLRP3, ASC, Caspase-1, IL1β and Actin were detected by western blot (e) and RT-PCR (f). The samples came from one mouse per experiment and results were representative of three independent experiments. NLRP3 expression levels were quantitated by measuring band intensities using ‘ImageJ’ software. The values were normalized to actin. **P<0.01. Mean and s.d. of three samples. Figure 1: AhR inhibits NLRP3 expression. ( a , b ) Mouse peritoneal macrophages were pretreated with dimethylsuphoxide (DMSO) or TCDD for 40 min and then stimulated with LPS for the indicated periods. NLRP3, ASC, caspase-1, IL1β and Actin were detected by western blot ( a ) and RT-PCR ( b ). ( c ) Mouse peritoneal macrophages were pretreated with increasing concentration of TCDD (2, 10, 20, 50 nM) or FICZ (20, 100, 200, 500 nM) for 40 min and then stimulated with LPS for 8 h. NLRP3 and Actin were detected by western blot. ( d ) Western blot analysis of NLRP3, ASC, Procaspase-1, AhR and Actin expression in mouse peritoneal macrophages transfected with scrambled control siRNA or AhR siRNA for 48 h. ( e , f ) Mouse peritoneal macrophages transfected with control siRNA or AhR siRNA were stimulated with LPS for the indicated periods. NLRP3, ASC, Caspase-1, IL1β and Actin were detected by western blot ( e ) and RT-PCR ( f ). The samples came from one mouse per experiment and results were representative of three independent experiments. NLRP3 expression levels were quantitated by measuring band intensities using ‘ImageJ’ software. The values were normalized to actin. ** P <0.01. Mean and s.d. of three samples. Full size image To investigate the function of AhR on LPS-induced NLRP3 expression under physiological conditions, two synthesized interfering RNAs (siRNA 1 and 2) targeting mouse AhR were used to suppress endogenous AhR expression. AhR knockdown greatly decreased AhR expression and enhanced NLRP3 expression in mouse peritoneal macrophages ( Fig. 1d ). AhR siRNA 2, which has a higher efficiency to inhibit AhR expression, has a greater potential to increase NLRP3 production ( Fig. 1d ). Therefore, AhR siRNA 2 was used in the following experiments. In addition, AhR knockdown significantly increased LPS-induced NLRP3 expression at both protein and mRNA level ( Fig. 1e,f ). We further investigated whether AhR inhibited NLRP3 expression at the transcription level. A murine NLRP3 promoter plasmid −2032 (nt −2032 to nt +166) was transiently transfected into RAW264.7 cells. LPS stimulation significantly induced the luciferase activity of NLRP3 and TCDD treatment greatly inhibited the NLRP3 promoter activation ( Fig. 2a ). Furthermore, other AhR agonists including FICZ and L -kynurenine treatment also greatly inhibited LPS-induced NLRP3 promoter activation ( Fig. 2b ). To examine the effect of AhR on NLRP3 promoter activation, we established a RAW264.7 cell line that stably expressed AhR (RAW-AhR) and RAW-Vector stably transfected with empty vector as control. As shown in Fig. 2c , LPS-induced NLRP3 promoter activation was significantly inhibited in RAW-AhR cells compared with that in RAW-Vector cells. Collectively, these data indicate that AhR inhibits NLRP3 expression at the transcription level. 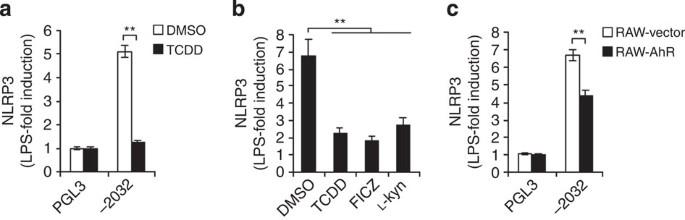Figure 2: AhR inhibits NLRP3 transcription. (a) RAW264.7 cells transfected with the NLRP3 promoter plasmids −2032 were pretreated with dimethylsuphoxide (DMSO) or TCDD for 40 min and then stimulated with LPS for 6 h. (b) RAW264.7 cells transfected with the NLRP3 promoter plasmids −2032 were pretreated with DMSO, TCDD, FICZ orL-kynurenine (L-kyn) for 40 min and then stimulated with LPS for 6 h. (c) RAW-AhR or RAW-Vector cells were transfected with the NLRP3 promoter plasmids −2032 and then stimulated with LPS for 6 h. The cell lysates were assayed for luciferase activity. The ratio of stimulated versus unstimulated activities is shown. **P<0.01. Data are representative of three experiments (mean and s.d. of six samples). Figure 2: AhR inhibits NLRP3 transcription. ( a ) RAW264.7 cells transfected with the NLRP3 promoter plasmids −2032 were pretreated with dimethylsuphoxide (DMSO) or TCDD for 40 min and then stimulated with LPS for 6 h. ( b ) RAW264.7 cells transfected with the NLRP3 promoter plasmids −2032 were pretreated with DMSO, TCDD, FICZ or L -kynurenine ( L -kyn) for 40 min and then stimulated with LPS for 6 h. ( c ) RAW-AhR or RAW-Vector cells were transfected with the NLRP3 promoter plasmids −2032 and then stimulated with LPS for 6 h. The cell lysates were assayed for luciferase activity. The ratio of stimulated versus unstimulated activities is shown. ** P <0.01. Data are representative of three experiments (mean and s.d. of six samples). Full size image AhR binds to NLRP3 promoter and inhibits NLRP3 transcription It has been reported that AhR controls the transcriptional activity of genes through direct binding to XRE in its target gene promoter [22] , [23] , [26] . On the basis of our findings that the AhR has a key role in the regulation of NLRP3 expression, we hypothesized that the AhR might bind to NLRP3 promoter and modulate its transcription activity. The XRE sequences consisting of conserved core sequences 5′- (A/T)NGCGTG -3′ are found in the regulatory regions of a variety of genes [22] . We then first searched the murine NLRP3 promoters and found three putative XREs: AGCTGCGTG (XRE-1: nt −1512 to −1504), TGCGCGTG (XRE-2: nt −911 to −904) and TATGCGTG (XRE-3: nt +60 to +67) ( Fig. 3a ). To confirm the function of these XREs in LPS-induced NLRP3 expression, various luciferase reporters with different length of NLRP3 promoter and XRE deletion (ΔXRE) or mutation (mt) reporters were constructed ( Fig. 3b ). 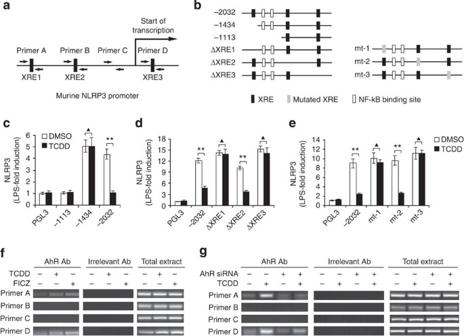Figure 3: AhR binds to NLRP3 promoter and inhibits NLRP3 transcription. (a) The potential AhR binding site in the murine NLRP3 promoter. Filled boxes, AhR-binding sites (XRE). Filled arrows, primers used for ChIP assay. (b) Schematic diagram of luciferase plasmids with different length of NLRP3 promoter, XRE deletion (ΔXRE) or mt. Open boxes, NF-κB binding sites. Grey filled boxes, mutated XRE. (c) RAW264.7 cells transfected with the NLRP3 promoter plasmids −2032, −1434 or −1113 were pretreated with dimethylsuphoxide (DMSO) or TCDD for 40 min and then stimulated with LPS for 6 h. (d) RAW264.7 cells transfected with the NLRP3 promoter mutants NLRP3 ΔXRE1, NLRP3 ΔXRE2 or NLRP3 ΔXRE3 were pretreated with DMSO or TCDD for 40 min and then stimulated with LPS for 6 h. (e) RAW264.7 cells transfected with the NLRP3 promoter mutants NLRP3 mt-1, NLRP3 mt-2, or NLRP3 mt-3 were pretreated with DMSO or TCDD for 40 min and then stimulated with LPS for 6 h. The cell lysates were assayed for luciferase activity. The ratio of stimulated versus unstimulated activities is shown. (f) Mouse peritoneal macrophages were pretreated with DMSO, TCDD or FICZ for 1 h, and the ChIP assay was used to assess the binding of AhR to the XRE in the murine NLRP3 promoter. (g) Mouse peritoneal macrophages transfected with control siRNA or AhR siRNA were pretreated with DMSO or TCDD for 40 min and then stimulated with LPS for 1 h, and the ChIP assay was used to assess the binding of AhR to the XRE in the murine NLRP3 promoter. Total extract was used as a loading control, and immunoprecipitation with irrelevant antibody (anti-actin) was used as a negative control. PCR products from the amplication of an AhR site-free region of the murine NLRP3 promoter were used as specificity controls. Similar results were obtained in three independent experiments. **P<0.01.▴, no significant differences. Data are representative of three experiments (mean and s.d. of triplicate samples inc–e). Figure 3: AhR binds to NLRP3 promoter and inhibits NLRP3 transcription. ( a ) The potential AhR binding site in the murine NLRP3 promoter. Filled boxes, AhR-binding sites (XRE). Filled arrows, primers used for ChIP assay. ( b ) Schematic diagram of luciferase plasmids with different length of NLRP3 promoter, XRE deletion (ΔXRE) or mt. Open boxes, NF-κB binding sites. Grey filled boxes, mutated XRE. ( c ) RAW264.7 cells transfected with the NLRP3 promoter plasmids −2032, −1434 or −1113 were pretreated with dimethylsuphoxide (DMSO) or TCDD for 40 min and then stimulated with LPS for 6 h. ( d ) RAW264.7 cells transfected with the NLRP3 promoter mutants NLRP3 ΔXRE1, NLRP3 ΔXRE2 or NLRP3 ΔXRE3 were pretreated with DMSO or TCDD for 40 min and then stimulated with LPS for 6 h. ( e ) RAW264.7 cells transfected with the NLRP3 promoter mutants NLRP3 mt-1, NLRP3 mt-2, or NLRP3 mt-3 were pretreated with DMSO or TCDD for 40 min and then stimulated with LPS for 6 h. The cell lysates were assayed for luciferase activity. The ratio of stimulated versus unstimulated activities is shown. ( f ) Mouse peritoneal macrophages were pretreated with DMSO, TCDD or FICZ for 1 h, and the ChIP assay was used to assess the binding of AhR to the XRE in the murine NLRP3 promoter. ( g ) Mouse peritoneal macrophages transfected with control siRNA or AhR siRNA were pretreated with DMSO or TCDD for 40 min and then stimulated with LPS for 1 h, and the ChIP assay was used to assess the binding of AhR to the XRE in the murine NLRP3 promoter. Total extract was used as a loading control, and immunoprecipitation with irrelevant antibody (anti-actin) was used as a negative control. PCR products from the amplication of an AhR site-free region of the murine NLRP3 promoter were used as specificity controls. Similar results were obtained in three independent experiments. ** P <0.01. ▴ , no significant differences. Data are representative of three experiments (mean and s.d. of triplicate samples in c – e ). Full size image Transcription factor NF-κB is critical for NLRP3 expression and two NF-κB binding sites in the NLRP3 promoter region from nt −1434 to −1113 are responsible for LPS-induced NLRP3 expression [10] , [27] . Consistent with these findings, we found that LPS stimulation significantly induced the luciferase activity of NLRP3 (−2032) and NLRP3 (−1434) reporters, but not of NLRP3 (−1113) reporter ( Fig. 3c ). TCDD treatment greatly inhibited the NLRP3 (−2032) promoter activation and had no effect on the NLRP3 (−1434) promoter activation in RAW264.7 cells ( Fig. 3c ). Furthermore, TCDD treatment inhibited the luciferase activity in the NLRP3 −2032 and NLRP3 ΔXRE-2 reporters, but lost its inhibitory effects in NLRP3 ΔXRE-1 and NLRP3 ΔXRE-3 reporter ( Fig. 3d ). Similarly, TCDD treatment inhibited the luciferase activity in the NLRP3 mt-2 reporters, but lost its inhibitory effects in NLRP3 mt-1 and NLRP3 mt-3 reporter ( Fig. 3e ). Collectively, these data indicated that XRE-1 and XRE-3 were both responsible for the AhR function. To investigate whether AhR can interact with its target sequences in the NLRP3 promoter, chromatin immunoprecipitation (ChIP) assays were performed. AhR could constitutively bind to the NLRP3 promoter region containing XRE-1 (nt −1588 to nt −1399) and XRE-3 (nt +36 to nt +161) and TCDD or FICZ treatment enhanced the DNA binding activity ( Fig. 3f ), whereas AhR could not bind to NLRP3 promoter regions containing XRE-2 (nt −962 to nt −841) and XRE-free region (nt −697 to nt −492) from the same setting of TCDD- or FICZ-stimulated macrophages, indicating specific binding of AhR to the promoter region containing XRE-1 and XRE-3. The presence of natural AhR agonists in culture medium (for example, DMEM or RPMI 1640) contribute to background AhR activation [28] , [29] and exogenous administration of TCDD or FICZ increases the activity of AhR. Furthermore, in AhR knockdown primary macrophages, AhR binding to the NLRP3 promoter was greatly decreased ( Fig. 3g ). Taken together, these results demonstrate that AhR binds to the NLRP3 promoter and negatively regulates NLRP3 expression. AhR inhibits NLRP3 inflammasome activation The sufficient NLRP3 protein expression is crucial for the formation and activation of NLRP3 inflammasome [8] , [9] . Given the fact that AhR negatively regulated NLRP3 expression, we tested whether AhR could inhibit NLRP3 inflammasome activation. As shown in Fig. 4a , TCDD treatment significantly decreased caspase-1 cleavage in LPS primed macrophages treated by Nigericin, ATP or Alum. Consistent with the AhR activation experiments, more cleaved caspase-1 was detected in AhR siRNA treated macrophages ( Fig. 4b ). Recent studies indicate that cotreatment with LPS and endogenous stress signals, (such as extracellular ATP) is sufficient for the rapid activation of NLRP3 inflammasome [30] , [31] , which is not dependent on NLRP3 upregulation. As shown in Fig. 4c , stimulation of macrophages with ATP and LPS for 30 min led to rapid caspase-1 activation and TCDD treatment had no effects on the caspase-1 activation. These data suggested that AhR activation negatively regulated NLRP3 inflammasome activation indirectly through its effects on NLRP3 transcription. 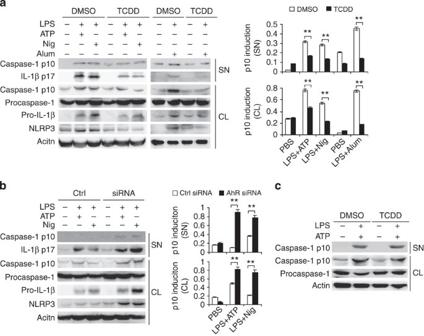Figure 4: AhR inhibits NLRP3 inflammasome. (a) Mouse peritoneal macrophages were pretreated with dimethylsuphoxide (DMSO) or TCDD for 40 min and then stimulated with LPS for 8 h and ATP, nigericin (Nig) or Alum for the last 30 min. (b) Mouse peritoneal macrophages transfected with scrambled control siRNA or AhR siRNA were stimulated with LPS for 8 h and ATP or nigericin (Nig) for the last 30 min. Western blot of cleaved caspase-1 (p10), cleaved IL-1β (p17), procaspase-1 and pro-IL-1β in the supernatants (SN) or cell lysates (CL). (c) Mouse peritoneal macrophages were pretreated with DMSO or TCDD for 40 min and then stimulated with LPS together with ATP for 30 min. Western blot of cleaved caspase-1 (p10) and procaspase-1. The samples came from one mouse per experiment and results were representative of three independent experiments. Cleaved caspase-1 (p10) expression levels were quantitated by measuring band intensities using ‘ImageJ’ software. The values were normalized to actin. **P<0.01. Mean and s.d. of three samples. Figure 4: AhR inhibits NLRP3 inflammasome. ( a ) Mouse peritoneal macrophages were pretreated with dimethylsuphoxide (DMSO) or TCDD for 40 min and then stimulated with LPS for 8 h and ATP, nigericin (Nig) or Alum for the last 30 min. ( b ) Mouse peritoneal macrophages transfected with scrambled control siRNA or AhR siRNA were stimulated with LPS for 8 h and ATP or nigericin (Nig) for the last 30 min. Western blot of cleaved caspase-1 (p10), cleaved IL-1β (p17), procaspase-1 and pro-IL-1β in the supernatants (SN) or cell lysates (CL). ( c ) Mouse peritoneal macrophages were pretreated with DMSO or TCDD for 40 min and then stimulated with LPS together with ATP for 30 min. Western blot of cleaved caspase-1 (p10) and procaspase-1. The samples came from one mouse per experiment and results were representative of three independent experiments. Cleaved caspase-1 (p10) expression levels were quantitated by measuring band intensities using ‘ImageJ’ software. The values were normalized to actin. ** P <0.01. Mean and s.d. of three samples. Full size image Activation of caspase-1 leads to the cleavage of pro-IL-1β and secretion of mature IL-1β. We then evaluated the effects of AhR on IL-β secretion. TCDD treatment significantly inhibited IL-1β secretion in a dose-dependent manner in macrophages ( Fig. 5a,b ). Other AhR agonists including FICZ and L -kynurenine also greatly inhibited IL-1β secretion ( Fig. 5c ). Furthermore, the overexpression of AhR resulted in decreased secretion of IL-1β ( Fig. 5d ). To investigate AhR inhibition of inflammasome activation under physiological conditions, endogenous AhR expression was knocked down by siRNA in mouse peritoneal macrophages and IL-1β secretion was measured. AhR knockdown resulted in augmented secretion of IL-1β, whereas AhR activation by TCDD treatment has an opposite effect ( Fig. 5e ). However, TCDD treatment had no effects on the IL-1β secretion in AhR siRNA transfected macrophages ( Fig. 5e ), indicating TCDD inhibited IL-1β secretion in an AhR-dependent manner. Collectively, these data indicate that AhR inhibits NLRP3 inflammasome activation and subsequent IL-1β production. 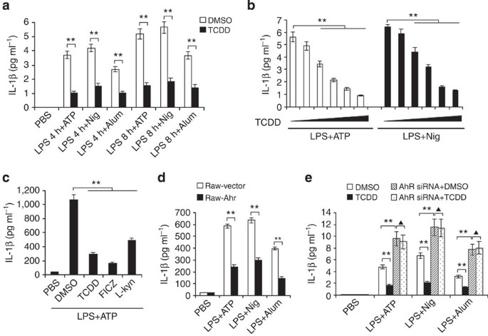Figure 5: AhR inhibits IL-1β secretion. (a) Mouse peritoneal macrophages were pretreated with dimethylsuphoxide (DMSO) or TCDD for 40 min and then stimulated with LPS for the indicated periods and ATP, nigericin (Nig) or Alum for the last 30 min. (b) Mouse peritoneal macrophages were pretreated with increasing concentration of TCDD (2, 10, 20, 50 nM) for 40 min and then stimulated with LPS for 8 h and ATP or nigericin (Nig) for the last 30 min. (c) Mouse peritoneal macrophages were pretreated with DMSO, TCDD, FICZ orL-kynurenine (L-kyn) for 40 min and then stimulated with LPS for 8 h and ATP or nigericin (Nig) for the last 30 min. The level of IL-1β in the culture supernatants was determined by ELISA. (d) RAW-Vector or RAW-AhR cells were stimulated with LPS for 8 h and ATP, nigericin (Nig) or Alum for the last 30 min. The level of IL-1β in the culture supernatants was determined by ELISA. (e) Mouse peritoneal macrophages transfected with scrambled control siRNA or AhR siRNA were pretreated with DMSO or TCDD for 40 min and then stimulated with LPS for 8 h and ATP, nigericin (Nig) or Alum for the last 30 min. The level of IL-1β in the culture supernatants was determined by ELISA. **P<0.01.▴, no significant differences. Data are representative of three experiments (mean and s.d. of triplicate samples). Figure 5: AhR inhibits IL-1β secretion. ( a ) Mouse peritoneal macrophages were pretreated with dimethylsuphoxide (DMSO) or TCDD for 40 min and then stimulated with LPS for the indicated periods and ATP, nigericin (Nig) or Alum for the last 30 min. ( b ) Mouse peritoneal macrophages were pretreated with increasing concentration of TCDD (2, 10, 20, 50 nM) for 40 min and then stimulated with LPS for 8 h and ATP or nigericin (Nig) for the last 30 min. ( c ) Mouse peritoneal macrophages were pretreated with DMSO, TCDD, FICZ or L -kynurenine ( L -kyn) for 40 min and then stimulated with LPS for 8 h and ATP or nigericin (Nig) for the last 30 min. The level of IL-1β in the culture supernatants was determined by ELISA. ( d ) RAW-Vector or RAW-AhR cells were stimulated with LPS for 8 h and ATP, nigericin (Nig) or Alum for the last 30 min. The level of IL-1β in the culture supernatants was determined by ELISA. ( e ) Mouse peritoneal macrophages transfected with scrambled control siRNA or AhR siRNA were pretreated with DMSO or TCDD for 40 min and then stimulated with LPS for 8 h and ATP, nigericin (Nig) or Alum for the last 30 min. The level of IL-1β in the culture supernatants was determined by ELISA. ** P <0.01. ▴ , no significant differences. Data are representative of three experiments (mean and s.d. of triplicate samples). Full size image AhR suppresses Alum-induced peritonitis in vivo We further investigated whether the biological effects of in vitro AhR activation on IL-1β production were similar in vivo using an IL-1-dependent mouse peritonitis model. Mouse peritonitis was induced by intraperitoneal (i.p.) injection of alum [14] , [17] . Peritoneal exudate cells (PECs) were collected and alum-induced recruitment of inflammatory cells was analysed by flow cytometry. As shown in Fig. 6a , alum challenge greatly upregulated mature IL-1β secretion in the lavage fluid and that this was significantly attenuated by TCDD or FICZ pretreatment, which was consistent with the observation in vitro . Furthermore, AhR activation also inhibited other proinflammatory cytokines production, such as tumour necrosis factor-α (TNF-α) and IL-6 ( Fig. 6b ). In addition, less caspase-1 cleavage was also observed in the lavage fluid from TCDD or FICZ pretreated mice ( Fig. 6c ). We consequently analysed alum-induced recruitment of inflammatory cells in the lavage fluid. Alum-induced recruitment of PECs was strongly reduced in the mice pretreated with TCDD or FICZ ( Fig. 6d ). Neutrophil and Ly6C + monocyte recruitment was also significantly blocked by TCDD or FICZ pretreatment ( Fig. 6d ). Collectively, these findings further demonstrated that AhR activation could inhibit NLRP3 inflammasome activity and subsequent immune cell accumulation in mouse peritonitis in vivo . 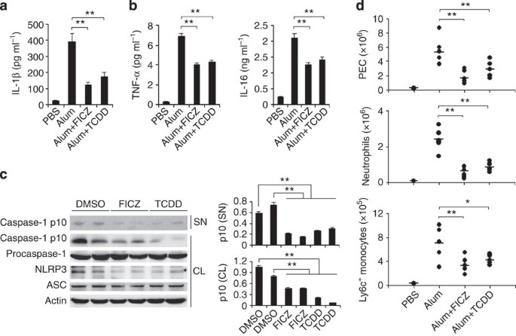Figure 6: AhR suppresses Alum-induced peritonitisin vivo. C57BL/6 mice were i.p. injected with dimethylsuphoxide (DMSO), TCDD or FICZ for 40 min, and then i.p. injected with Alum for 12 h. (a,b) IL-1β, TNF-α and IL-6 content in the lavage fluid was measured by ELISA (six mice per group). (c) PECs recovered were lysed and analysed for their expression of caspase-1 and NLRP3 by immunoblot. Cleaved caspase-1 (p10) expression levels were quantitated by measuring band intensities using ‘ImageJ’ software. The values were normalized to actin. **P<0.01. Mean and s.d. of three samples. (d) Absolute numbers of PECs, neutrophils or Ly6C+monocytes recruited to the peritoneum were analysed by fluorescence-activated cell sorting (six mice per group). **P<0.01, *P<0.05. Data are representative of three experiments. Figure 6: AhR suppresses Alum-induced peritonitis in vivo . C57BL/6 mice were i.p. injected with dimethylsuphoxide (DMSO), TCDD or FICZ for 40 min, and then i.p. injected with Alum for 12 h. ( a , b ) IL-1β, TNF-α and IL-6 content in the lavage fluid was measured by ELISA (six mice per group). ( c ) PECs recovered were lysed and analysed for their expression of caspase-1 and NLRP3 by immunoblot. Cleaved caspase-1 (p10) expression levels were quantitated by measuring band intensities using ‘ImageJ’ software. The values were normalized to actin. ** P <0.01. Mean and s.d. of three samples. ( d ) Absolute numbers of PECs, neutrophils or Ly6C + monocytes recruited to the peritoneum were analysed by fluorescence-activated cell sorting (six mice per group). ** P <0.01, * P <0.05. Data are representative of three experiments. Full size image AhR plays important roles in the differentiation and function of multiple types of immune cells such as T cells, macrophages, dendritic cells and so on [22] , [23] , [24] . For example, various AhR ligands such as TCDD regulate the differentiation of Treg cells and Th17 cells [26] , [32] , [33] , [34] , and modulate Th1/Th2 balance [35] . AhR in combination with STAT1 negatively regulates proinflammatory cytokine production by inhibiting NF-κB activation in macrophages after LPS stimulation [25] . AhR knockout mice are hypersensitive to LPS-induced septic shock, mainly due to macrophage dysfunction [36] . AhR interacts with RORγt, promotes AhR binding at the IL-22 locus and promotes the development of RORγt + innate lymphoid cells [37] . AhR mediates the above-mentioned immunoregulatory roles mainly via regulation of various genes’ expression including IL-10, IL-21, IL-22, TNF-α, IL-6 and Foxp3. AhR could directly bind to the promoter region of its target genes and modulate their transcription. In addition to its activation effects on target genes, the repression role of AhR has also been reported [38] , [39] , [40] . For example, AhR mediated inhibition of 17β-Estradiol (E2)-induced cathepsin D gene expression is due to AhR binding to the XRE region located between the ER and Sp1 response elements and disrupting the ER-Sp1 complex with an overlapping XRE [38] . AhR binds to the XRE located in the pS2 promoter region and interacts with AP-1-like proteins, which may be responsible for TCDD-mediated inhibition of E2-induced pS2 expression [39] . AhR complex interacted with the XRE that also overlapped the E2-responsive GC-rich site in the c-fos gene promoter, and that may quench or mask the Sp1-binding site, leading to the suppression of E2-induced c-fos expression [40] . Consistent with these reports, we found that AhR could bind to XRE (−1512 to −1504 and +60 to +67) in the NLRP3 promoter on AhR activation and then inhibit NLRP3 transcription in macrophages ( Fig. 7 ). 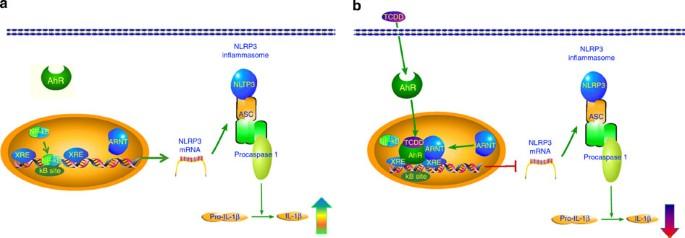Figure 7: Proposed model illustrating how AhR negatively regulates NLRP3 inflammasome activation. (a) NF-κB binds to the κB site located in the promoter of NLRP3 and initiates the gene expression. NLRP3 then promotes the formation of NLRP3 inflammasome, leading to the cleavage of procaspase-1. Active caspase-1 then promotes the cleavage of pro-IL-1β and secretion of mature IL-1β. (b) Following engagement by its cognate ligands, eg TCDD, AhR forms a heterodimer with ARNT in nucleus, binds to the XRE regions located at the two sides of κB site in the promoter of NLRP3 and inhibits NF-κB transcription activity, resulted in the decrease of NLRP3 transcription and subsequent inflammasome activation. Figure 7: Proposed model illustrating how AhR negatively regulates NLRP3 inflammasome activation. ( a ) NF-κB binds to the κB site located in the promoter of NLRP3 and initiates the gene expression. NLRP3 then promotes the formation of NLRP3 inflammasome, leading to the cleavage of procaspase-1. Active caspase-1 then promotes the cleavage of pro-IL-1β and secretion of mature IL-1β. ( b ) Following engagement by its cognate ligands, eg TCDD, AhR forms a heterodimer with ARNT in nucleus, binds to the XRE regions located at the two sides of κB site in the promoter of NLRP3 and inhibits NF-κB transcription activity, resulted in the decrease of NLRP3 transcription and subsequent inflammasome activation. Full size image NF-κB is critical for NLRP3 expression and two NF-κB binding sites in the NLRP3 promoter region (−1434 to −1113) are responsible for LPS-induced NLRP3 transcription [10] , [27] . We also found that LPS stimulation could not induce NLRP3 luciferase activity in NLRP3 (−1113) reporter ( Fig. 3c ), which bears no functional NF-κB binding sites. AhR complex interacted with the XRE regions located at the two sides of NF-κB binding sites ( Fig. 3f ), and the association may block NF-κB DNA binding or mask the NF-κB transcription activity, leading to the inhibition of NLRP3 expression. The inhibitory effects of AhR on NF-κB transcription activity has been well demonstrated [41] , [42] . AhR may suppress NF-κB activity in a competition model or associate with AhR in a ‘tethered’ manner, and then prevent transcriptional processes [42] , [43] . Furthermore, it has been reported that AhR complex binding to the promoter of target genes may alter high-order chromatin structure and gene expression is then attenuated [44] . AhR may attenuate NLRP3 transcription in such a manner. The precise mechanisms for AhR inhibition of NLRP3 gene transcription are under investigation. Typically, AhR forms a heterodimer with ARNT in the nucleus and AhR–ARNT complex modulates transcription of genes with promoters containing XRE consensus sequence. Besides the ‘classical’ pathway of AhR, the non-canonical interactions between AhR and RelA, STAT1 are important for the biological functions of AhR. For example, AhR agonists have been shown to repress or transactivate NF-κB response genes [22] , [42] , [43] , [44] , [45] . The interaction between AhR and STAT1 is relevant for the abrogation of STAT1 signalling and subsequent Th17 differentiation [46] . The activated AhR and NF-κB are both capable of binding to coactivator complexes, p300/CBP and SRC-1, which are required for full transcription of either pathway [41] , [47] . By competing for coactivators of one pathway may cause transrepression of the other pathway [41] . This type of scenario has also been proposed for the inhibitory effects of AP-1 and STAT1 (refs 48 , 49 ). AhR inhibited LPS-induced expression of proinflammatory cytokines (for example, IL-6, TNF-α) through suppressing NF-κB transcriptional activity together with STAT1 (ref. 25 ). Consistently, we found that AhR activation inhibited LPS-mediated pro-IL-1β expression at both the protein and mRNA levels ( Fig. 1a,b ), and AhR knockdown had the opposite effects ( Fig. 1e,f ). Caspase-1-mediated cleavage of pro-IL-1β is critical for secretion of mature IL-1β. In the present study, we found that AhR inhibited NLRP3 inflammasome formation, caspase-1 activation and subsequent IL-1β secretion. Thus, AhR may inhibit IL-1β production at multiple levels including suppression of NLRP3 inflammasome activation and NF-κB activity. On the basis of the experimental data discussed above, we propose a model to illustrate how AhR could negatively regulate the NLRP3 expression and subsequent inflammasome activation ( Fig. 7 ). NLRP3 is the rate-limiting element for the activation of inflammasome. It has been reported that the activation status of NLRP3 inflammasome resulted from NLRP3 expression level is highly correlated with multiple diseases, such as autoinflammatory syndromes, metabolic diseases and cancers. Thus, tight control of the NLRP3 expression is critical for the prevention of these diseases. In the present study, our work defines AhR as a negative regulator of NLRP3 expression at the transcriptional level. Considering the ubiquitous abundance of AhR ligands in food and environmental pollutants, this suppression effect may commonly exist and cause defective activity of NLRP3 inflammasome. Disturbance of the function of NLRP3 inflammasome may further compromise cellular integrity. Thus, our research provides a molecular pathway by which the environment can affect the immune response and the development of immune-mediated disorders. Furthermore, our results also provide a strategy to downregulate inflammasome activity and suggest that AhR may constitute a potential target for the therapeutic modulation of sterile inflammatory diseases such as autoinflammatory diseases, atherosclerosis, obesity and diabetes. Mice, cells and reagents C57BL/6J mice were obtained from Joint Ventures Sipper BK Experimental Animal (Shanghai, China). All animal experiments were undertaken in accordance with the National Institute of Health Guide for the Care and Use of Laboratory Animals, with the approval of the Scientific Investigation Board of Medical School of Shandong University, Jinan, Shandong Province, China. To obtain mouse primary peritoneal macrophages, C57BL/6J mice (female, 4–6-week old) were injected i.p. with 3% Brewer’s thioglycollate broth. Three days later, PEC were collected and incubated. Two hours later, nonadherent cells were removed and the adherent monolayer cells were used as peritoneal macrophages. Mouse macrophage cell line RAW264.7 cells were obtained from American Type Culture Collection (Manassas, VA). The cells were cultured at 37 °C under 5% CO 2 in DMEM supplemented with 10% FCS (Invitrogen-Gibco), 100 U ml −1 penicillin and 100 μg ml −1 streptomycin [50] , [51] . ATP, nigericin, L -kynurenine and LPS (Escherichia coli, 055:B5) were from Sigma-Aldrich (St Louis, MO); TCDD was from Cambridge Isotope Laboratories (Woburn, MA, USA); Imject Alum (77161) was from Thermo Scientific; FICZ, anti-NLRP3 Ab and anti-ASC Ab were from Enzo Life Sciences (Farmingdale, NY); anti-AhR Ab (ab2770) was from Abcam (Cambridge, MA); anti-IL-1β Ab was from Cell Signaling Technology (Beverly, MA); anti-caspase-1 p10 Ab and anti-actin Ab were from Santa Cruz Biotechnology (Santa Cruz, CA). The concentration of agonists or stimuli were used as below: LPS 100 ng ml −1 , TCDD 10 nM, FICZ 100 nM, L -kynurenine 25 μM, ATP 2 mM, nigericin 50 μM and Alum 200 μg ml −1 . Sequences, plasmid constructs and transfection The murine NLRP3 promoter plasmids −2032 (nt −2032 to nt +166), −1434 (nt −1434 to nt +166) and −1113 (nt −1113 to nt +166) were described before [27] . In NLRP3 ΔXRE-1, NLRP3 ΔXRE2 and NLRP3 ΔXRE3 reporter plasmids, the intact XRE (GCGTG) was deleted. In NLRP3 mt-1, NLRP3 mt-2 and NLRP3 mt-3 reporter plasmids, the GCGTG was mutated to ATACA. All the NLRP3 promoter mutants were generated from the NLRP3-2032 promoter plasmid using the KOD-Plus-Mutagenesis kit (Toyobo). AhR cDNA was amplified from mouse primary peritoneal macrophages by PCR and cloned in pCMV-Myc plasmid. All constructs were confirmed by DNA sequencing. For transient silencing, duplexes of small interfering RNA were transfected into cells with the Geneporter 2 Transfection Reagent (GTS, San Diego) according to the standard protocol. Target sequences for transient silencing were 5′- GAGGAACCUUGGGAUUGAU -3′ (siRNA 1) and 5′- GAGGGAUUAACUUCUAGAU -3′ (siRNA 2) for AhR, ‘scrambled’ control sequences were 5′- UUCUCCGAACGUGUCACGU -3′. For transient transfection of plasmids into RAW264.7 cells, jetPEI reagents were used (Polyplus transfection). For stable selection of RAW264.7 cell lines overexpressing AhR, transfected RAW264.7 macrophages were selected with G418 (800 μg ml −1 ) and pooled for further experiments. ELISA The concentrations of IL-1β, TNF-α and IL-6 were measured using ELISA kits (Dakewe Biotech Company Ltd., Shenzhen, China) according to the manufacturer’s instruction. RT-PCR and western blot Total RNA was extracted with TRIzol reagent according to the manufacturer’s instructions (Invitrogen). The sequences of primers used for reverse transcription-PCR (RT-PCR) were 5′- TGGATGGGTTTGCTGGGAT -3′ and 5′- CTGCGTGTAGCGACTGTTGAG -3′ for NLRP3; 5′- CTGGAGTCGTATGGCTTGGAG -3′ and 5′- CAAAGTGTCCTGTTCTGGCTGTA -3′ for ASC; 5′- TTGAAAGACAAGCCCAAGGTG -3′ and 5′- CTGGTGTTGAAGAGCAGAAAGC -3′ for Caspase-1; 5′- ACCTTCCAGGATGAGGACATGA -3′ and 5′- AACGTCACACACCAGCAGGTTA -3′ for IL-1β; 5′- TGTTACCAACTGGGACGACA -3′ and 5′- CTGGGTCATCTTTTCACGGT -3′ for β-actin. Three independent RT-PCR data are presented as Supplementary Fig. 4 . For western blot, cells were lysed with M-PER Protein Extraction Reagent (Pierce, Rockford, IL) supplemented with a protease inhibitor ‘cocktail’, then protein concentrations in the extracts were measured with a bicinchoninic acid assay (Pierce, Rockford, IL). Equal amounts of extracts were separated by SDS-polyacrylamide gel electrophoresis, and then were transferred onto nitrocellulose membranes for immunoblot analysis [50] , [51] . Scans of the full films used to generate western blot data and another two replicates are presented as Supplementary Figs 1–3 . NLRP3 or caspase-1 p10 expression levels were quantitated by measuring band intensities using ‘ImageJ’ software. The values were normalized to actin. Luciferase assay Luciferase activities were measured with Dual-Luciferase Reporter Assay System (Promega) according to the manufacturer’s instructions [50] , [51] . Data are normalized for transfection efficiency by subtracting Firefly luciferase activity with that of Renilla luciferase. ChIP assay Chromatin from macrophages was fixed and immunoprecipitated using the ChIP assay kit (Upstate Biotechnology, Inc.) according to the manufacturer’s instructions [52] . The purified chromatin was immunoprecipitated using 2 μg of anti-AhR or irrelevant antibody (anti-actin). The presence of the selected DNA sequence was assessed by PCR. The primers were 5′- AGCCTGACAGGTGAGACCAAAA -3′, 5′- GACATAAGCAGTGGCAAGCAGA -3′ for NLRP3 promoter (−1588 to −1399); 5′- GGGATGTTCTGTTTGCTGTTACG -3′, 5′- TGCCACCCTGAGTAGATGCTG -3′ for NLRP3 promoter (−962 to −841); 5′- GACACGAGTCCTGGTGACTTTG -3′, 5′- TCCAGACGTATGTCCTGAGCC -3′ for NLRP3 promoter (−697 to −492); and 5′- AAAGTCTAGGAGGATCTGTGGAGC -3′, 5′- GAAAGTGCCTGAAAGGTGGTG -3′ for NLRP3 promoter (+36 to +161). The average size of the sonicated DNA fragments subjected to immunoprecipitation was 500 bp as determined by ethidium bromide gel electrophoresis. In vivo peritonitis C57BL/6J mice (females, 6-week old) were i.p. injected with dimethylsulphoxide, 50 μg kg −1 TCDD or 200 μg kg −1 FICZ for 40 min, and then i.p. injected with 700 μg Alum for 12 h. Peritoneal cavities were washed with 6 ml of PBS. The peritoneal fluids were collected and concentrated for ELISA analysis with Amicon Ultra 10K from Millipore. Peritoneal exudates cells (PECs) were analysed by fluorescence-activated cell sorting [14] , [17] . Statistical analysis All experiments were independently performed three times. Data are presented as means±s.d. of three or four experiments. Analysis was performed using a Student’s t -test or analysis of variance. Values of P <0.05 were considered to be statistically significant. How to cite this article: Huai, W. et al . Aryl hydrocarbon receptor negatively regulates NLRP3 inflammasome activity by inhibiting NLRP3 transcription. Nat. Commun. 5:4738 doi: 10.1038/ncomms5738 (2014).